Perceptual judgements and chronic imaging of altered odour maps indicate comprehensive stimulus template matching in olfaction Lesion experiments suggest that odour input to the olfactory bulb contains significant redundant signal such that rodents can discern odours using minimal stimulus-related information. Here we investigate the dependence of odour-quality perception on the integrity of glomerular activity by comparing odour-evoked activity maps before and after epithelial lesions. Lesions prevent mice from recognizing previously experienced odours and differentially delay discrimination learning of unrecognized and novel odour pairs. Poor recognition results not from mice experiencing an altered concentration of an odour but from perception of apparent novel qualities. Consistent with this, relative intensity of glomerular activity following lesions is altered compared with maps recorded in shams and by varying odour concentration. Together, these data show that odour recognition relies on comprehensively matching input patterns to a previously generated stimulus template. When encountering novel odours, access to all glomerular activity ensures rapid generation of new templates to perform accurate perceptual judgements. Establishing the relation between stimulus-evoked activity and sensory perception is central to determining how neuronal networks construct internal representations of the external world. To examine this question, in vivo chronic imaging has proven useful for assessing the large-scale spatial dynamics of network response properties [1] , [2] and for quantifying changes in those responses to sensory deprivation [1] , [3] , [4] , [5] or enrichment [6] , [7] . In parallel, behavioural and lesion experiments have been implemented to elucidate the psychophysical properties of sensory processing and the biological loci and function of neuronal elements involved [8] , [9] , [10] , [11] . In the olfactory system, glomeruli in the olfactory bulb receive stimulus-related information from olfactory receptor neurons (ORNs) expressing the same receptor that is then processed and integrated by bulbar circuitry [12] , [13] , [14] , [15] . The principal mitral and tufted cells that participate in glomerular circuits relay the resultant signals to olfactory cortex, where it is suggested that olfactory object templates [16] , [17] and odour-related memories [18] , [19] , [20] , [21] , [22] , [23] may be generated and stored. In the bulb, monomolecular odorants are known to evoke specific spatiotemporal activation sequences of glomeruli [24] , [25] , [26] , [27] ; however, the relevance of specific patterns of glomerular activity to odour quality perception has been a long-standing question. Both optical imaging [28] , [29] , [30] , [31] , [32] , [33] and high-resolution 2-deoxy-glucose studies of the bulb [24] , [34] , [35] indicate that although patterns of glomerular activation vary across both species and individuals [33] , the neuronal representation of odour quality is reflected by activity in distinct bulbar regions, indicative of a broad odotopic organization [36] . However, these glomerular patterns are widely distributed [24] , [29] , [31] , [33] , reflecting the activation of many different ORN types by even simple monomolecular odorants. Behavioural experiments on the other hand indicate that much of the widespread bulbar activation may not be required for olfactory perceptual judgements. Partial bulb lesions have been shown to have little or no impact on the discrimination of even highly similar odorants [10] , [11] . Moreover, in extreme cases, where rodents have undergone double bulbectomies, and thus abolition of all glomerular-based information, newly generated ORNs that extend their axons through the cribriform plate and form contacts in the forebrain are sufficient to support odour detection and discrimination of odorants [37] . Thus, extensive disruption of glomerular activity maps is believed to have very little or no effect on odour quality perception, indicating that such maps contain substantial redundant information that is not used for odour-related decision making [10] , [38] . Understanding the impact of altering odour-evoked activity on odour perception can yield information about the neuronal mechanisms the olfactory system relies on to determine the identity of an odour. Recent functional magnetic resonance imaging studies in humans [16] , [39] have provided evidence for models where the olfactory system uses preformed odour templates to match a stimulus to a previously experienced odour [40] . To directly test the idea of sensory redundancy and stimulus template matching in olfaction we combined chronic functional imaging of the olfactory bulb in mice with a non-surgical epithelial lesion that alters the ORN inputs that generate glomerular activity maps [41] . This allowed us to quantify differences in functional activity maps in mice where sensory inputs to the olfactory bulb are disrupted. Psychophysical assessment of odour quality perception in these mice shows that subtle changes in odour-evoked glomerular activity impairs recognition of familiar odours and impacts the time-course of discrimination learning of novel odours compared with previously experienced odours. These effects cannot be explained by perceived reductions in odour concentration or an increased detection threshold following lesioning. Rather, we conclude that all available glomerular information is used to generate a detailed reference template and that matching glomerular activity to that template ensures accurate, rapid olfactory-related decision making. Effects of ZnSO 4 -induced lesions on odour recognition Mice were first trained to accurately discriminate monomolecular odorants [10] , [18] , [42] (for example, amyl-acetate versus cineol; pair A discrimination task: Supplementary Figs S1 and S2 ) followed by a second odour pair (pair B discrimination task; ethyl-butyrate versus pentanal, Fig. 1a ). After performing above criterion for pair B odours, mice were tested for recognition of odour pair A by interleaving unrewarded pair A odour trials with pair B discrimination trials (pair A recognition test, Fig. 1b , Supplementary Fig. S2c ). Mice could recognize pair A odours with high accuracy, as pair A recognition test scores were not significantly different from the average of the last five blocks of pair A discrimination (pair A discrimination, 93.97±0.67% versus recognition 92.23%±1.89, P >0.19, n =14 mice). 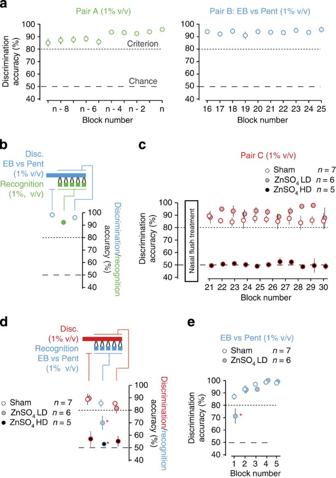Figure 1: Odour discrimination and recognition following nasal epithelial lesioning. (a) Left: discrimination scores (n=18 mice) obtained for the final ten blocks of training on pair A odours (green open circles), before presentation of a novel odour pair (pair B). Right: discrimination scores obtained for the final ten blocks of training on pair B odours (blue open circles). (b) Recognition scores of familiar pair A odours (green filled circles,n=14 mice). Also plotted are the discrimination scores for pair B odours for the block of trials immediately before (left blue circle) and those trials presented during recognition testing (indicated by thin blue lines,n=14 mice). (c) Discrimination scores obtained for the last ten blocks of training on novel pair C odours for sham (open circles), low-dose ZnSO4-treated (grey-filled circles) and high-dose ZnSO4-treated mice (black-filled circles). (d) Recognition scores for previously presented pair B odours (blue circles). Also plotted are the discrimination scores for pair C odours (red circles) for the block of trials immediately preceding and those trials presented during recognition testing (indicated by thin red lines). (e) Discrimination scores for previously presented pair B odours in sham and low-dose ZnSO4-treated mice presented immediately after recognition testing. Pair A odours were amyl acetate, cineol or eugenol. Pair B odours were ethyl butyrate and pentanal. Pair C odours were eugenol, limonene, valeric acid, heptanone or cineol. Data represent mean±s.e.m. *P<0.02 (one-tailed two sample Student’st-tests). Figure 1: Odour discrimination and recognition following nasal epithelial lesioning. ( a ) Left: discrimination scores ( n =18 mice) obtained for the final ten blocks of training on pair A odours (green open circles), before presentation of a novel odour pair (pair B). Right: discrimination scores obtained for the final ten blocks of training on pair B odours (blue open circles). ( b ) Recognition scores of familiar pair A odours (green filled circles, n =14 mice). Also plotted are the discrimination scores for pair B odours for the block of trials immediately before (left blue circle) and those trials presented during recognition testing (indicated by thin blue lines, n =14 mice). ( c ) Discrimination scores obtained for the last ten blocks of training on novel pair C odours for sham (open circles), low-dose ZnSO 4 -treated (grey-filled circles) and high-dose ZnSO 4 -treated mice (black-filled circles). ( d ) Recognition scores for previously presented pair B odours (blue circles). Also plotted are the discrimination scores for pair C odours (red circles) for the block of trials immediately preceding and those trials presented during recognition testing (indicated by thin red lines). ( e ) Discrimination scores for previously presented pair B odours in sham and low-dose ZnSO 4 -treated mice presented immediately after recognition testing. Pair A odours were amyl acetate, cineol or eugenol. Pair B odours were ethyl butyrate and pentanal. Pair C odours were eugenol, limonene, valeric acid, heptanone or cineol. Data represent mean±s.e.m. * P <0.02 (one-tailed two sample Student’s t -tests). Full size image Mice were then briefly anaesthetized with isoflurane and treated in one of three ways; with 0.9% w/v NaCl (sham), with a ‘low dose’ of ZnSO 4 (three nasal flushes of 8.4% w/v ZnSO 4 per naris) or a ‘high dose’ (2 × three nasal flushes per naris of 8.4% w/v ZnSO 4 ). Following a 24-h recovery period, mice were given 30 blocks of training in which to learn to discriminate a new odour pair (pair C). Once they reached criterion, performance of mice treated with a low dose of ZnSO 4 was not significantly different from shams (last block of pair C discrimination task, sham, 88.93±4.40%, n =7 versus low-dose ZnSO 4 , 89.66±2.86%, n =6, P >0.44, Fig. 1c ). High-dose ZnSO 4 -treated mice, however, discriminated at chance levels on pair C odours for all 30 blocks (all 30 blocks, 49.93±0.69%, χ 2 -test significance from 50%, n =5 mice, P >0.82. Last five blocks, 49.66±1.31%, P >0.26, Fig. 1c ). Mice were next tested for recognition of the pretreatment pair B odours. Despite their accurate discrimination of pair C odours, low-dose ZnSO 4 -treated animals returned subcriterion recognition scores that were on average significantly lower than shams (shams, 85.7±2.97%, n =7; low-dose ZnSO 4 , 70±5.47%, n =6, P <0.02; Fig. 1d ) that is not explained by rapid extinction in the low-dose group ( Supplementary Fig. S3 ). For recognition, high-dose-ZnSO 4 -treated mice performed at chance levels, with recognition scores that were significantly lower than both shams and low-dose-ZnSO 4 -treated mice (53.00±1.22%, n =5 mice versus shams, P <0.0001, versus low-dose-ZnSO 4 -treated, P <0.013). To ensure that low-dose-ZnSO 4 -treated mice could detect the previously experienced pair B odours, their ability to relearn to discriminate this odour pair (with the S+ odour rewarded again) was assessed. Although low-dose-ZnSO 4 -treated mice initially performed significantly worse than shams (first block, sham 87±2.45%, n =7 mice versus low-dose-ZnSO 4 -treated, 71.25±6.06%, n =6 mice, P <0.01), they quickly reached criterion on pair B odours (second block, sham, 92.86±3.25%, n =7 mice versus low-dose-ZnSO 4 -treated, 92.5±2.92%, n =6 mice, P >0.46; Fig. 1e ), indicating that they could detect and discriminate the previously experienced pretreatment odours. Effects of lesions on glomerular activity maps We next recorded intrinsic signals evoked by the recognition test odours (ethyl-butyrate and pentanal) from the dorsal surface of the bulb before (imaging session one) and following (imaging session two) nasal flush treatment (see Methods and Supplementary Fig. S4 ). Qualitatively, although the integrity of the odour-evoked glomerular map was maintained for sham-treated mice, low-dose-ZnSO 4 -treated mice revealed a phenotype ranging from very minor map changes to an almost complete abolition of odour-evoked signals. In no mice receiving the high-dose ZnSO 4 treatment did we detect odour-evoked signals (0/9 mice tested for two odours). To quantify the effect of low-dose ZnSO 4 treatment on map activity, pixel intensity values of regions of interest (ROI) were correlated with the concomitant ROI recorded in activity maps evoked by the same odour in the same olfactory bulb ( Supplementary Fig. S5 ). Correlation coefficients for each ROI were compared between maps recorded in the same session to generate a within-session correlation value and between maps recorded in different sessions to produce an across-session correlation value ( Fig. 2a ). Across-session correlations were subtracted from within-session correlations, yielding a dissimilarity score whereby high scores indicate large differences between session one and session two activity maps. Although signals from sham-treated animals had low dissimilarity scores (0.104±0.03, n =27 activity maps), mice treated with a low dose of ZnSO 4 showed significantly higher dissimilarity scores (0.340±0.05, n =32 odour-evoked activity maps, P <0.0002, Fig. 2c ). Mice treated with the high dose of ZnSO 4 showed significantly higher dissimilarity scores than both sham- and low-dose-ZnSO 4 -treated animals, consistent with signal abrogation in these animals (0.573±0.07, n =16 odour-evoked activity maps, versus sham, P <10 −5 , versus low-dose ZnSO 4 , P <0.005, data not shown). 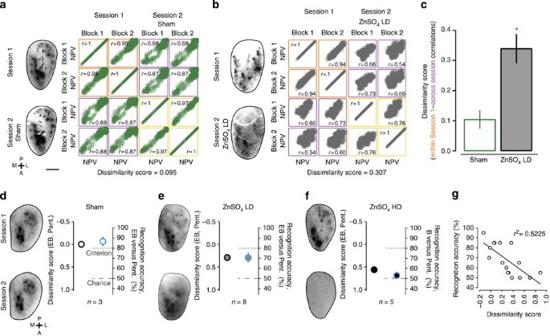Figure 2: Effects of epithelial lesioning on odour-evoked intrinsic optical images and odour recognition. (a) Example scatter plots of ROI correlations for odour-evoked intrinsic signal activity maps recorded within sessions (session one, orange boxes; session two, yellow boxes) and across sessions (purple boxes) after sham treatment. Values for each ROI (open green circles) are expressed as normalized pixel value (NPV),r-values displayed are averages of all ROI correlations for each block comparison. The total number of data points plotted correspond to nROIs × pixels/ROI for one odour. Concomitant activity maps are displayed to the left of NPV correlations. NPV range, 0.9965–1.0027. Scale bar, 500 μm for all images. (b) Example scatter plots of ROI correlations (grey) for odour-evoked intrinsic signal activity maps within sessions (session one, orange boxes; session two, yellow boxes) and across sessions (purple boxes) after low-dose ZnSO4treatment. (c) Bar graph showing dissimilarity score of intrinsic signal activity maps (evoked by ethyl-butyrate and pentanal) from sham (n=27 activity maps, green open box) and low-dose-ZnSO4-treated animals (n=32 activity maps, grey-filled box). NPV range, 0.996302−1.000254. Dissimilarity scores evaluated by Mann–WhitneyU-test (*P<0.001). (d) Left, example odour-evoked activity maps from before (top, session one) and after (bottom, session two) nasal flush for sham-treated mice. Right, average dissimilarity score for pair B odour-evoked activity maps (left axis) and recognition scores for pair B odours (right axis) for shams. (e,f) As above for low- (e) and high-dose (f) ZnSO4-treated mice. Data represent mean±s.e.m. (g) Recognition accuracy plotted against dissimilarity score for ethyl butyrate and pentanal from all mice in D1–D3. Pearson’s correlation value,P<0.05. Figure 2: Effects of epithelial lesioning on odour-evoked intrinsic optical images and odour recognition. ( a ) Example scatter plots of ROI correlations for odour-evoked intrinsic signal activity maps recorded within sessions (session one, orange boxes; session two, yellow boxes) and across sessions (purple boxes) after sham treatment. Values for each ROI (open green circles) are expressed as normalized pixel value (NPV), r -values displayed are averages of all ROI correlations for each block comparison. The total number of data points plotted correspond to nROIs × pixels/ROI for one odour. Concomitant activity maps are displayed to the left of NPV correlations. NPV range, 0.9965–1.0027. Scale bar, 500 μm for all images. ( b ) Example scatter plots of ROI correlations (grey) for odour-evoked intrinsic signal activity maps within sessions (session one, orange boxes; session two, yellow boxes) and across sessions (purple boxes) after low-dose ZnSO 4 treatment. ( c ) Bar graph showing dissimilarity score of intrinsic signal activity maps (evoked by ethyl-butyrate and pentanal) from sham ( n =27 activity maps, green open box) and low-dose-ZnSO 4 -treated animals ( n =32 activity maps, grey-filled box). NPV range, 0.996302−1.000254. Dissimilarity scores evaluated by Mann–Whitney U -test (* P <0.001). ( d ) Left, example odour-evoked activity maps from before (top, session one) and after (bottom, session two) nasal flush for sham-treated mice. Right, average dissimilarity score for pair B odour-evoked activity maps (left axis) and recognition scores for pair B odours (right axis) for shams. ( e , f ) As above for low- ( e ) and high-dose ( f ) ZnSO 4 -treated mice. Data represent mean±s.e.m. ( g ) Recognition accuracy plotted against dissimilarity score for ethyl butyrate and pentanal from all mice in D1–D3. Pearson’s correlation value, P <0.05. Full size image In a subset of mice, we were able to perform behavioural assessment, epithelial lesions and chronic imaging to determine the dependence of recognition on dissimilarity score ( Fig. 2d-f ). Sham-treated mice had, on average, both significantly higher recognition scores and lower dissimilarity scores than low-dose-ZnSO 4 -treated mice (pair B recognition scores, shams, 86.6±4.41%, n =3 versus low-dose-ZnSO 4 -treated, 70.6±4.67%, n =8 mice, P <0.05; pair B dissimilarity scores, shams, −0.0378±0.04, n =10 activity maps versus low-dose-ZnSO 4 -treated, 0.29±0.07, n =21 activity maps, P <0.02). High-dose-ZnSO 4 -treated mice also had significantly lower recognition and higher dissimilarity scores than both sham- and low-dose-ZnSO 4 -treated mice (pair B recognition scores, 53±1.37%, n =5 versus shams, P <0.001, versus low-dose-ZnSO 4 -treated, P <0.003. Pair B dissimilarity scores 0.56±0.07, n =15 activity maps versus shams, P <0.02, versus low-dose-ZnSO 4 -treated, P <0.02, Fig. 2d–f ). The overall correlation between the dissimilarity and recognitions scores for ethyl butyrate and pentanal in this subset of animals was also significant ( r 2 =0.53, P <0.05, n =16 mice, 47 maps) ( Fig. 2g ). We interpret these initial observations in the following way; first, as mice receiving high-dose ZnSO 4 treatment could neither discriminate pair C odours nor recognize pair B odours, and showed no detectable odour-evoked intrinsic signal activity, they were likely anosmic (at least for the odour pairs tested). Second, low-dose ZnSO 4 treatment caused a significant alteration in ORN activity that is accompanied by a significant reduction in ability to recognize previously experienced odours, and likely reflects an altered percept of those odorants. Recognition of familiar odours at novel concentrations One possible alternative explanation for the recognition scores in the low-dose-ZnSO 4 -treated group could be that treatment induces a homogeneous reduction in ORN input, resulting in an odorant being perceived at an apparent lower concentration during recognition testing. Although rodents have been shown to extrapolate odour identity over ~10-fold changes in concentration [43] , larger changes in concentration can cause them to respond as though odours appear in some way novel, that is, with reduced foraging times in associative tasks [44] . To therefore test the possibility that low-dose-ZnSO 4 -treated mice recognize previously experienced odours but do not generalize across concentrations on this task, a group of naive mice were first trained on pair A and then on pair B odours all presented at 1% v/v ( Fig. 3a ). Lower concentrations (0.05 or 0.01% v/v) of pair A odours were presented for the recognition test ( Fig. 3b ). Indeed, when test odours were reduced in concentration 20- to 100-fold from the trained pair A odour, average recognition scores were significantly lower than for control animals probed with odours presented at the previously experienced concentration of 1% v/v (1% v/v, 92.14±3.02%, n =7 versus 0.05% v/v, 78.13±7.07%, n =8, P <0.047; 0.01% v/v, 71.67±11.67, n =3, P <0.03, Fig. 3b ). 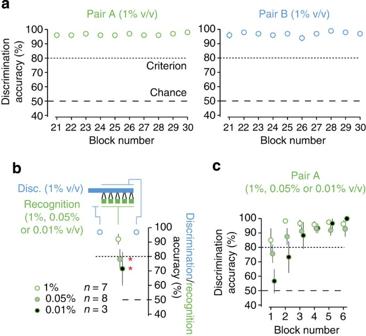Figure 3: Recognition of novel concentrations of previously presented odours. (a) Left, Discrimination scores (n=18 mice) obtained for each of the final ten blocks of training on pair A odours (green open circles), before presentation of a novel odour pair (pair B). Right, discrimination scores obtained for the final ten blocks of training on pair B odours (blue open circles). (b) Recognition scores (green circles) for mice tested with previously presented concentrations of pair A odours (1% v/v, open circles) and pair A odours at novel concentrations (0.05% v/v, grey-filled circles; 0.01% v/v, black-filled circles). Also plotted are the discrimination scores for pair B odours (blue circles) at previously presented concentrations for the block of trials immediately preceding and those trials presented during recognition testing (indicated by thin blue lines). (c) Discrimination scores for previously presented pair A odours at novel concentrations presented immediately following recognition testing. Pair A odours were ethyl butyrate and pentanal. In the 0.05% v/v group,n=2 were amyl acetate and cineol. Pair B odours were amyl acetate, cineol, ethyl butyrate, pentanal or eugenol. Data represent mean±s.e.m. *P<0.05 (one-tailed two sample Student’st-tests). Figure 3: Recognition of novel concentrations of previously presented odours. ( a ) Left, Discrimination scores ( n =18 mice) obtained for each of the final ten blocks of training on pair A odours (green open circles), before presentation of a novel odour pair (pair B). Right, discrimination scores obtained for the final ten blocks of training on pair B odours (blue open circles). ( b ) Recognition scores (green circles) for mice tested with previously presented concentrations of pair A odours (1% v/v, open circles) and pair A odours at novel concentrations (0.05% v/v, grey-filled circles; 0.01% v/v, black-filled circles). Also plotted are the discrimination scores for pair B odours (blue circles) at previously presented concentrations for the block of trials immediately preceding and those trials presented during recognition testing (indicated by thin blue lines). ( c ) Discrimination scores for previously presented pair A odours at novel concentrations presented immediately following recognition testing. Pair A odours were ethyl butyrate and pentanal. In the 0.05% v/v group, n =2 were amyl acetate and cineol. Pair B odours were amyl acetate, cineol, ethyl butyrate, pentanal or eugenol. Data represent mean±s.e.m. * P <0.05 (one-tailed two sample Student’s t -tests). Full size image Again, to ensure mice could detect the low concentration recognition test odours, they were retrained to discriminate pair A odours at the reduced concentration ( Fig. 3c ). The first and second blocks of pair A discrimination scores were significantly lower in mice presented with 0.01% v/v (second block, 1% v/v, 98.33±1.67%, n =7 versus 0.01% v/v, 73.33±10.93%, n =3, P <0.007) but were then indistinguishable from controls (third block, 1% v/v, 96.67±2.47% versus 0.01% v/v, 88.33±9.28%, P >0.13). Discrimination scores for odours presented at 0.05% v/v were not significantly different from 1% v/v odours on the first block of discrimination training trials (1% v/v, 85.00±8.16% versus 0.05% v/v, 75.63±6.43%, P >0.17). Together, these data suggest that on this Go/No-Go task, mice trained to discriminate monomolecular odorants at a single concentration later respond to the same odour when presented at 20- to 100-fold lower concentration as though it is being perceived in some way different. The effect of concentration training on recognition We therefore next sought to train mice on a range of odour concentrations so that presentation of an unfamiliar, low concentration of the same odour may be responded to as being familiar. Following the successful discrimination of ethyl butyrate and pentanal at concentrations of 0.01, 0.1, 0.25 and 1% v/v (now pair A odours; Fig. 4a–d ), mice were trained to discriminate pair B odours at 1% v/v ( Fig. 4e ). Once they reached criterion on pair B odours, unfamiliar concentrations of ethyl butyrate and pentanal (0.05% v/v) were presented as the recognition test odours. After concentration training, mice achieved above criterion recognition scores for unfamiliar low concentrations of ethyl butyrate and pentanal, indistinguishable from those scores obtained from mice presented with the familiar 1% v/v concentration (1% v/v, 91.67±2.79%, n =6 versus 0.05% v/v, 97.14±2.14%, n =7, P >0.07, Fig. 4f ). Furthermore, recognition of 0.05% v/v odours following concentration pretraining was significantly higher than for recognition of 0.05% v/v odours in mice without concentration training (0.05%, v/v, without training, 78.13±7.07%, n =8; 0.05% v/v, trained, 97.14±2.14%, n =7, P <0.01). 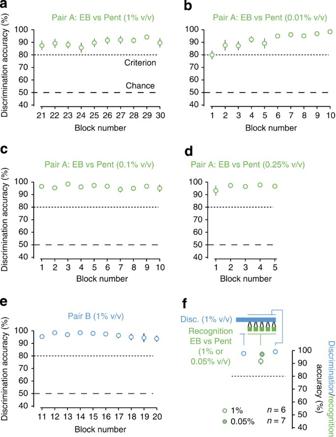Figure 4: Recognition of novel concentrations following concentration training. (a–d) Discrimination scores (n=13 mice) obtained for each of the final ten blocks of training on pair A odours at 1% v/v (a). Discrimination scores obtained for the first ten blocks of training on pair A odours at concentrations of 0.01% v/v (b), 0.1% v/v (c) and 0.25% v/v (d). (e) Discrimination scores obtained for the final ten blocks of training on pair B odours at 1% v/v. (f) Recognition scores (green circles) for mice presented with familiar concentrations of pair A odours (1% v/v, open circles) or pair A odours at novel concentrations (0.05% v/v, grey-filled circles). Also plotted are the discrimination scores for pair B odours (blue circles) for the block of trials immediately preceding and those trials presented during recognition testing (indicated by thin blue lines). Pair A odours were ethyl butyrate and pentanal, pair B odours were eugenol and cineol. Data represent mean±s.e.m. Figure 4: Recognition of novel concentrations following concentration training. ( a – d ) Discrimination scores ( n =13 mice) obtained for each of the final ten blocks of training on pair A odours at 1% v/v ( a ). Discrimination scores obtained for the first ten blocks of training on pair A odours at concentrations of 0.01% v/v ( b ), 0.1% v/v ( c ) and 0.25% v/v ( d ). ( e ) Discrimination scores obtained for the final ten blocks of training on pair B odours at 1% v/v. ( f ) Recognition scores (green circles) for mice presented with familiar concentrations of pair A odours (1% v/v, open circles) or pair A odours at novel concentrations (0.05% v/v, grey-filled circles). Also plotted are the discrimination scores for pair B odours (blue circles) for the block of trials immediately preceding and those trials presented during recognition testing (indicated by thin blue lines). Pair A odours were ethyl butyrate and pentanal, pair B odours were eugenol and cineol. Data represent mean±s.e.m. Full size image If low-dose ZnSO 4 treatment results in recognition test odours being perceived as though presented at a reduced concentration, then pre-training low-dose-ZnSO 4 -treated mice on a range of concentrations would be expected to improve recognition scores, as demonstrated above. However, despite being trained to discriminate a range of concentrations (0.01, 0.1, 0.25 and 1% v/v) of ethyl butyrate and pentanal ( Fig. 5a–f ), and being able to learn to discriminate pair C odours (shams, 96.75±1.35%, n =5, low-dose-ZnSO 4 -treated, 96.67±2.47%, P >0.48), low-dose-ZnSO 4 -treated animals continued to perform below criterion for recognition of ethyl butyrate and pentanal (presented at 1% v/v) and were significantly worse than shams (sham, 1% v/v, 96.00±1.87%, n =5 versus low-dose ZnSO 4 , 1% v/v, 65.00±8.56%, n =6, P <0.008, Fig. 5g ). Again, to determine whether low-dose-ZnSO 4 -treated mice retained the ability to detect the unrecognized odours, mice were retrained to discriminate this odour pair (at 1% v/v). As above, although low-dose-ZnSO 4 -treated mice initially performed significantly worse than shams, they quickly learned to discriminate unrecognized odours within two blocks (first block, sham, 93.00±3.74% versus low-dose-ZnSO 4 -treated, 64.17±8.89%, P <0.02; second block, sham, 97.00±2.00% versus low-dose-ZnSO 4 -treated, 89.17±8.00%, P >0.2, Fig. 5h ). Relearning of discrimination of unrecognized odours was also not significantly different between concentration trained and non-concentration-trained low-dose-ZnSO 4 -treated mice (first five blocks, block by block Student’s t -tests, all comparisons, all P -values: P >0.12; F (1,58) =1.7, P >0.19, Fig. 5i ). This data thus suggests that low-dose ZnSO 4 treatment alters apparent odour identity rather than its perceived concentration. 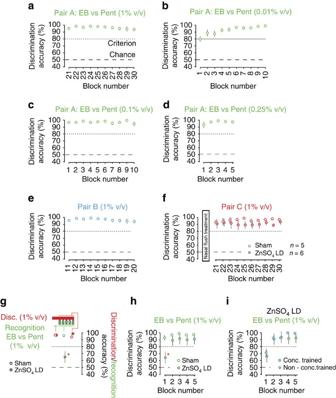Figure 5: Recognition of familiar odours in nasal–epithelial lesioned mice following concentration training. (a–d) Discrimination scores (n=11 mice) obtained for each of the final ten blocks of training on pair A odours at 1% v/v (a). Discrimination scores obtained for the first ten blocks of training on pair A odours at concentrations of 0.01% v/v (b), 0.1% v/v (c) and 0.25% v/v (d). (e) Discrimination scores obtained for the final ten blocks of training on pair B odours at 1% v/v. (f) Discrimination scores obtained for the last ten blocks of training on novel pair C odours for sham-treated (open circles) and low-dose-ZnSO4-treated mice (grey-filled circles). (g) Recognition scores for pair A odours (green circles) previously presented at a range of concentrations. Also plotted are the discrimination scores for pair C odours (red circles) for the block of trials immediately preceding and those trials presented during recognition testing (indicated by thin red lines). (h) Discrimination scores for previously presented pair A odours in sham and low-dose-ZnSO4-treated mice presented immediately following recognition testing. (i) Discrimination scores for previously presented pair A or B odours presented immediately following recognition testing. Plotted are scores for low-dose-ZnSO4-treated mice that were concentration trained (green, gray-filled circles) and non-concentration trained (blue, gray-filled circles). Pair A odours were ethyl butyrate and pentanal, pair B odours were eugenol and cineol, pair C odours were amyl acetate and limonene. Data represent mean±s.e.m. *P<0.05 (one-tailed two sample Student’st-tests). Figure 5: Recognition of familiar odours in nasal–epithelial lesioned mice following concentration training. ( a – d ) Discrimination scores ( n =11 mice) obtained for each of the final ten blocks of training on pair A odours at 1% v/v ( a ). Discrimination scores obtained for the first ten blocks of training on pair A odours at concentrations of 0.01% v/v ( b ), 0.1% v/v ( c ) and 0.25% v/v ( d ). ( e ) Discrimination scores obtained for the final ten blocks of training on pair B odours at 1% v/v. ( f ) Discrimination scores obtained for the last ten blocks of training on novel pair C odours for sham-treated (open circles) and low-dose-ZnSO 4 -treated mice (grey-filled circles). ( g ) Recognition scores for pair A odours (green circles) previously presented at a range of concentrations. Also plotted are the discrimination scores for pair C odours (red circles) for the block of trials immediately preceding and those trials presented during recognition testing (indicated by thin red lines). ( h ) Discrimination scores for previously presented pair A odours in sham and low-dose-ZnSO 4 -treated mice presented immediately following recognition testing. ( i ) Discrimination scores for previously presented pair A or B odours presented immediately following recognition testing. Plotted are scores for low-dose-ZnSO 4 -treated mice that were concentration trained (green, gray-filled circles) and non-concentration trained (blue, gray-filled circles). Pair A odours were ethyl butyrate and pentanal, pair B odours were eugenol and cineol, pair C odours were amyl acetate and limonene. Data represent mean±s.e.m. * P <0.05 (one-tailed two sample Student’s t -tests). Full size image Effects of odour concentration and lesioning on activity maps If low-dose ZnSO 4 treatment results in a previously presented odorant being perceived as novel and not merely reduced in concentration, one would expect the glomerular activity map altered by low-dose ZnSO 4 treatment to be changed in a manner that does not reflect map changes observed by varying odour concentrations. First, we tested this assumption by using correlations to compare intrinsic signal maps evoked by S+ and S− odours presented at varying concentrations. Intrinsic-signal activity maps recorded at 1% v/v odour concentrations in session one were compared with various concentrations recorded in session two. Over the range of concentrations recorded, dissimilarity scores for maps evoked by 1% v/v odours in session one and those evoked by varying odour concentrations in session two were not significantly different from dissimilarity scores for maps evoked by 1% v/v odour presentation in both sessions ( Supplementary Fig. S6 ). Activity maps were next analysed to determine whether low-dose ZnSO 4 treatment altered the intensity of ROIs relative to one another (see Supplementary Methods ). For all odour-evoked activity maps that contained ROI activity, we observed no reliable changes in the relative intensities of ROIs across concentrations (1% v/v session one−1% v/v session two, interquartile range=0.20, n =7; session two, 0.1% v/v, 0.17, n =5, P >0.60; session two, 0.05%v/v, 0.19, n =7, P >0.97; session two, 0.01% v/v, 0.25, n =7, P >0.83, Fig. 6d ). This is entirely consistent with experiments that show relative glomerular intensity remains constant over a moderate range of concentrations [34] , [44] , [45] , [46] , [47] . In contrast, low-dose ZnSO 4 treatment produced a marked change in relative ROI intensity across sessions compared with that of shams (sham, interquartile range Q1–Q3=0.24, n =15 versus low-dose ZnSO 4 treatment, 0.48, n =9, P <0.0004, Fig. 7a–g ). 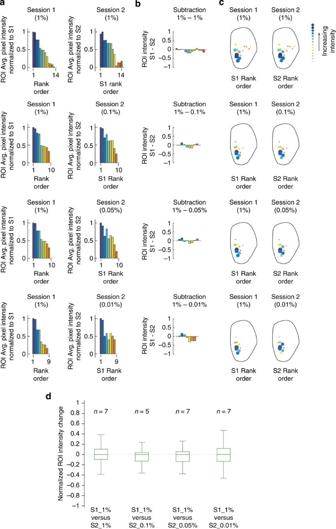Figure 6: Effects of varying odour concentrations on ROI intensities. (a) Left, example bar graphs of ranked average pixel intensity for each ROI evoked in session one by 1% v/v odours. ROI intensity is normalized to the maximum ROI in session one. Right, example bar graph of ranked average pixel intensity for each ROI evoked in session two by either 1, 0.1, 0.05 or 0.01% v/v odours. ROI intensity is normalized to the maximum ROI from session two. (b) Subtraction of session two ROI intensity values from session one values. (c) Average ROI pixel intensity map; large blue spots have the highest average pixel intensity, small, orange spots have the lowest average pixel intensity. Change in average pixel intensity rank between session one (left) and session two (right) is indicated by change of size and colour of an ROI spot. (d) Normalized ROI intensity change for subtraction values of all ROIs. Medians have been normalized to 0. Boxes indicate the first (bottom) and third (top) quartile. Whiskers extend to the most extreme data values within the range q1–1.5 × (q3–q1) to q3+1.5 × (q3–q1), where q1 and q3 are the 25th and 75th percentiles, respectively. Figure 6: Effects of varying odour concentrations on ROI intensities. ( a ) Left, example bar graphs of ranked average pixel intensity for each ROI evoked in session one by 1% v/v odours. ROI intensity is normalized to the maximum ROI in session one. Right, example bar graph of ranked average pixel intensity for each ROI evoked in session two by either 1, 0.1, 0.05 or 0.01% v/v odours. ROI intensity is normalized to the maximum ROI from session two. ( b ) Subtraction of session two ROI intensity values from session one values. ( c ) Average ROI pixel intensity map; large blue spots have the highest average pixel intensity, small, orange spots have the lowest average pixel intensity. Change in average pixel intensity rank between session one (left) and session two (right) is indicated by change of size and colour of an ROI spot. ( d ) Normalized ROI intensity change for subtraction values of all ROIs. Medians have been normalized to 0. Boxes indicate the first (bottom) and third (top) quartile. Whiskers extend to the most extreme data values within the range q1–1.5 × (q3–q1) to q3+1.5 × (q3–q1), where q1 and q3 are the 25th and 75th percentiles, respectively. 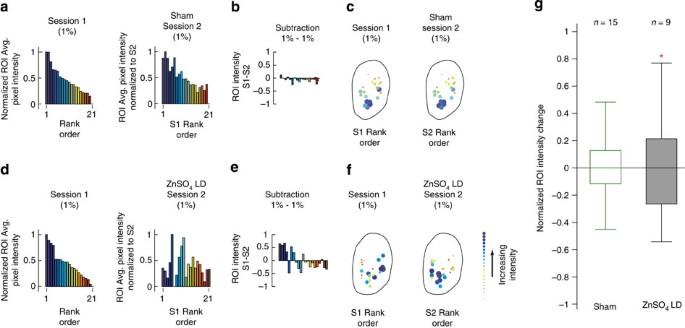Figure 7: Effects of nasal–epithelial lesioning on ROI intensities. (a) Left, example bar graph of ranked average pixel intensity for each ROI evoked in session one (S1). ROI intensity is normalized to the maximum ROI in session one. Right, example bar graph of ranked average pixel intensity for each ROI evoked in session two (S2). ROI intensity is normalized to the maximum ROI from session two. (b) Subtraction of session two ROI intensity values from session one values. (c) Average ROI pixel intensity map; large blue spots have the highest average pixel intensity, small, orange spots have the lowest average pixel intensity. Change in average pixel intensity rank between session one (left) and session two (right) is indicated by change of size and colour of an ROI spot. (d–f) Example as above for activity maps recorded in sessions 1 and 2 from a low-dose-ZnSO4-treated animal. (g) Normalized ROI intensity change for subtraction values of all ROIs. Medians have been normalized to 0. Boxes indicate the first (bottom) and third (top) quartile. Whiskers extend to the most extreme data values within the range q1–1.5 × (q3–q1) to q3+1.5 × (q3–q1), where q1 and q3 are the 25th and 75th percentiles, respectively. *P<0.001 (Ansari Bradley test of distribution). Full size image Figure 7: Effects of nasal–epithelial lesioning on ROI intensities. ( a ) Left, example bar graph of ranked average pixel intensity for each ROI evoked in session one (S1). ROI intensity is normalized to the maximum ROI in session one. Right, example bar graph of ranked average pixel intensity for each ROI evoked in session two (S2). ROI intensity is normalized to the maximum ROI from session two. ( b ) Subtraction of session two ROI intensity values from session one values. ( c ) Average ROI pixel intensity map; large blue spots have the highest average pixel intensity, small, orange spots have the lowest average pixel intensity. Change in average pixel intensity rank between session one (left) and session two (right) is indicated by change of size and colour of an ROI spot. ( d – f ) Example as above for activity maps recorded in sessions 1 and 2 from a low-dose-ZnSO 4 -treated animal. ( g ) Normalized ROI intensity change for subtraction values of all ROIs. Medians have been normalized to 0. Boxes indicate the first (bottom) and third (top) quartile. Whiskers extend to the most extreme data values within the range q1–1.5 × (q3–q1) to q3+1.5 × (q3–q1), where q1 and q3 are the 25th and 75th percentiles, respectively. * P <0.001 (Ansari Bradley test of distribution). Full size image The effect of lesions on odour discrimination To establish the degree of congruence between the sham and low-dose treatment groups in their ability to learn to discern odours, we pooled data from concentration- and non-concentration-trained mice to first assess whether there was an overall impact on the number of trials (that is, exposures) required to achieve criterion for (i) novel (pair B) odours before treatment, (ii) novel (pair C) odours after treatment and (iii) previously experienced but no longer recognized ethyl butyrate versus pentanal odours after treatment. Before treatment, there was no significant difference between the discrimination scores during discrimination training for novel pair B odours (repeated measures analysis of variance (ANOVA) for the first five blocks, shams versus low-dose-ZnSO 4 -treated, F (1,4) =0.8, P >0.52, Fig. 8a ). This was also the case when block scores from treated animals were aligned to the first block when shams, on average, reached criterion ( Fig. 8b ). However, for discrimination learning of novel set C odours ZnSO 4 -treated mice performed significantly and consistently worse than shams for the first 20 blocks (ANOVA, F (1,19) =3.49, P <10 −4 , Fig. 8c ) requiring more trials to reach criterion ( n =12 shams, n =12 low-dose-ZnSO 4 -treated mice, Fig. 8d ). 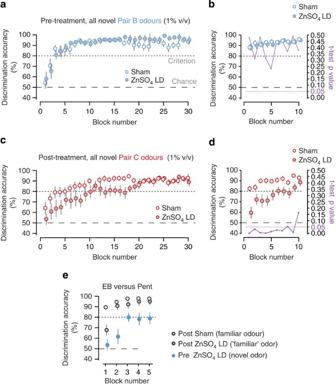Figure 8: Effects of ZnSO4 treatment on discrimination of novel and previously experienced odours. (a) Average pretreatment discrimination scores for sham-treated (n=12 mice, open circles) and low-dose-ZnSO4-treated mice (n=12 mice, grey-filled circles) for the first 30 blocks of novel pair B odour (1% v/v) discrimination training. (b) Discrimination learning for pair B odours plotted according to the first block when shams reached criterion (within each training group). Below are the respectiveP-values fort-tests performed between shams and low-dose-ZnSO4-treated groups for each block. (c) Average post-treatment discrimination scores for sham-treated (n=12 mice, open circles) and low-dose-ZnSO4-treated mice (n=12 mice, grey-filled circles) for the first 30 blocks of novel pair C odour (1% v/v) discrimination training. (d) Discrimination learning for pair C odours plotted according to the first block when shams reached criterion (within each training group). Below are the respectiveP-values for Student’st-tests performed between shams and low-dose-ZnSO4-treated groups for each block. (e) Discrimination learning scores for novel (1% v/v) ethyl butyrate (EB) and pentanal (Pent) presented before lesioning (blue filled circles). Also plotted are the post-treatment discrimination learning scores for EB and Pent for low-dose-ZnSO4-treated (grey filled circles) and shams (open circles). Figure 8: Effects of ZnSO4 treatment on discrimination of novel and previously experienced odours. ( a ) Average pretreatment discrimination scores for sham-treated ( n =12 mice, open circles) and low-dose-ZnSO 4 -treated mice ( n =12 mice, grey-filled circles) for the first 30 blocks of novel pair B odour (1% v/v) discrimination training. ( b ) Discrimination learning for pair B odours plotted according to the first block when shams reached criterion (within each training group). Below are the respective P -values for t -tests performed between shams and low-dose-ZnSO 4 -treated groups for each block. ( c ) Average post-treatment discrimination scores for sham-treated ( n =12 mice, open circles) and low-dose-ZnSO 4 -treated mice ( n =12 mice, grey-filled circles) for the first 30 blocks of novel pair C odour (1% v/v) discrimination training. ( d ) Discrimination learning for pair C odours plotted according to the first block when shams reached criterion (within each training group). Below are the respective P -values for Student’s t -tests performed between shams and low-dose-ZnSO 4 -treated groups for each block. ( e ) Discrimination learning scores for novel (1% v/v) ethyl butyrate (EB) and pentanal (Pent) presented before lesioning (blue filled circles). Also plotted are the post-treatment discrimination learning scores for EB and Pent for low-dose-ZnSO 4 -treated (grey filled circles) and shams (open circles). Full size image In low-dose-ZnSO 4 -treated animals, discrimination of previously experienced but not recognized odours (ethyl butyrate versus pentanal) was initially impaired compared with shams, but improved quickly (first block, shams, 89.5±2.20%, n =12, low-dose-ZnSO 4 -treated, 67.71±5.06%, n =12, P <0.001; second block, shams, 94.58±2.08%, low-dose-ZnSO 4 -treated, 90.83±4.35%, P >0.22, Fig. 8e ). Despite not accurately recognizing ethyl butyrate and pentanal, the post-treatment discrimination scores for these odours over the first five blocks were significantly improved compared with the scores for the same odours presented before treatment (ANOVA, F (1,118) =12.68, P <0.0005, Fig. 8e ). Thus, after lesioning ZnSO 4 -treated mice require more trials than shams to reach criterion on novel odours, but their discrimination relearning of the unrecognized ethyl butyrate versus pentanal pair is significantly better than for their initial training period on the same odour pair before lesioning. Taken together, our data show that low-dose ZnSO 4 treatment of the epithelium causes maps to be altered sufficiently such that previously experienced odours are not recognized. Despite being altered, these odour maps remain similar enough to pretreatment maps such that previously encountered odours may be ‘relearned’ and discerned more quickly than genuine novel odours. In contrast to previous studies [10] , [48] , [49] we have combined chronic functional imaging with peripheral olfactory epithelial lesions to directly examine the relationship between glomerular map functionality and odour-quality perception. We show that treatment of the epithelium with two different doses of ZnSO 4 results in two distinct olfactory behavioural phenotypes. High-dose treatment prevents recognition and discrimination of both familiar and novel odours. In support of this observation, we find no detectable odour-evoked signals on the dorsal surface of the olfactory bulb, consistent with an anosmic phenotype [50] , [51] . Low-dose ZnSO 4 treatment, on the other hand, resulted in mice that could not recognize previously presented odours, although they could detect and eventually learn to discriminate both previously presented and novel odour pairs. In contrast to the high dose, our intrinsic-signal imaging data revealed that low-dose ZnSO 4 treatment results in a modest functional alteration of the glomerular map. This suggests that the coding requirements for correct odour discrimination and recognition are sensitive to relatively minor changes to input patterns that is in contrast to previous suggestions [10] , [52] . One parsimonious explanation for our observations could be that low-dose ZnSO 4 treatment simply results in a homogenous reduction in the strength of input to the bulb. In this scenario, low-dose ZnSO 4 treatment would impair recognition by causing previously presented odours to be perceived at a novel, reduced concentration. Alternatively, ZnSO 4 treatment may cause mice to perceive previously presented odours as having distinctly unique qualities. In agreement with others [43] , [44] , [53] , our results show that in untreated mice trained on single concentrations, large differences in the training versus test odour concentration can cause mice to respond as if test odours appear in some way novel. We show that this is not the case when naive mice are pretrained on a series of test odour concentrations. However, despite being concentration pretrained, low-dose-ZnSO 4 -treated mice do not recognize familiar odours presented at familiar concentrations. Consistent with the notion that ZnSO 4 treatment alters odour perception in a way that is different to changing concentration, we observed significant differences in the relative intensity of glomerular activity compared with sham treatment and the effect of changing odour concentration. Previous studies focusing on the presynaptic ORN activity have reported that the relative intensity of glomerular activation is stable across a moderate range of odour concentrations similar to those used in both our imaging and behavioural experiments [45] , [47] . Conversely, axon tracing studies in the rat have shown that moderate nasal ZnSO 4 irrigation results in irregular sparing of glomerular innervation by ORNs, with the glomeruli receiving substantial numbers of spared axons intermingled with those receiving sparse or no innervation [52] . We therefore suggest that the non-homogenous effect of low-dose ZnSO 4 treatment on map activity impacts the integrity of the glomerular representation such that odour-quality perception is significantly impaired. Previous studies in mouse show that the regenerative process following complete ORN transection results in substantial miswiring between the receptor neuron axon and the target glomerulus [54] . Several months after transection when this regenerative process is completed, deficits in odour recognition have been observed in the hamster [55] . In our study we have assessed odour perception and map integrity within ten days post treatment, well before ORNs are believed to regenerate [50] , [56] . Although low-dose ZnSO 4 treatment perturbs input to the bulb, significant glomerular activity is spared. We find that this rather arbitrary manipulation impairs olfactory performance, whereby treated mice require significantly more trials to learn to discern novel odours compared with shams. In the case of previously presented odours not recognized after treatment, the impact of ZnSO 4 treatment on their discriminability is more subtle. Low-dose-ZnSO 4 -treated mice discriminate with the same accuracy as shams already after only one block of training. This rapid relearning of non-recognized odours is indeed faster than for the learning curve observed for mice when they are first exposed to the same odour pair before lesioning. This observation shows that after lesioning, the olfactory system does not process the unrecognized and novel odours in entirely the same way. The fact that low-dose-treated mice learn to discern non-recognized odours more quickly than novel odours indicates that odour stimulus templates stored before treatment remain relevant to the non-recognized odours and may be rapidly modified and used during post-treatment retraining. Along these lines, theoretical models suggest that predictive neuronal codes generated in advance of a stimulus [40] , [57] , [58] enhance the speed and accuracy of perceptual judgements. In this model, a pre-existing odour template and incoming sensory information interact to rapidly generate a sensory percept [40] , [42] . In accordance with our results, recent behavioural and/or imaging experiments indicate that activity patterns in piriform cortex may be the locus of such odour stimulus templates [16] , [17] . In summary, we show for the first time that perceptual correlates of odour concentration and other elements of odour identity are separable in rodents. We use this paradigm to determine that the effects of nasal–epithelial lesion with moderate concentrations of ZnSO 4 differ from reduction in concentration in that such lesions induce a unique change in the relative intensity of glomerular maps. Our data contrast previous work, indicating widespread lesions of the bulb have little or no impact on odour quality perception that has led to the suggestion that the spatially organized input to the bulb contains significant redundant information [10] , [11] , [48] , [59] . Our results support theoretical work and functional magnetic resonance imaging studies in humans that show that a cortical prestimulus template is used by the olfactory system to match incoming odour information to perform accurate perceptual judgements. We show that even relatively modest deviations from these templates can cause previously experienced odour stimuli not to be recognized. This suggests that coding in the olfactory bulb is non-redundant and that significant amounts of all available information is acquired to generate and match templates to perform rapid and accurate olfactory perceptual judgements. Animals All procedures and experiments were carried out on male C57Bl/6 mice over the ages of 4 weeks, in accordance with the UK Home Office and the Animals and Scientific Procedures Act, 1986. Behavioural training Mice were given restricted access to water for 48 h before behavioural training. After habituation to the olfactometer environment, they were trained to discriminate between two odours. Infrared beam interruption triggered presentation of either an S+ (reward coupled) or S− (unrewarded) odour. Lick patterns were recorded for the duration of the stimulus across four 350 ms time bins ( Supplementary Fig. S2a , top). Responses were deemed correct if the mouse licked for three or more time bins during presentation of the S+ odour, or if they licked for two or fewer time bins during the S− odour. Between 8 and 12 S+ and 12 and 8 S− odour trials were presented in a pseudo random order in blocks of 20 trials. Percentage of correct responses for S+ and S− trials was averaged over 20 trials, giving an overall percentage for each block ( Supplementary Fig. S2a , bottom). The mouse was classed as discriminating correctly when the average of each of five consecutive blocks first reached a criterion (≥80% correct, Supplementary Fig. S2b ). Mice usually performed between 20 and 30 blocks. Those mice trained on a range of concentrations were first trained to discriminate pair A odours at a concentration of 1% v/v. Next, pair A odours at lower concentrations were interleaved among higher concentrations forming pseudo blocks constituting, for example, 5S+ trials of 0.01% v/v, 5S+ trials of 1% v/v, 5S− 0.01% v/v trials and 5S− 1v/v% trials. Discrimination accuracy scores for two consecutive blocks were then averaged yielding full blocks (20 trials) of 10S+ and 10S− trials for both high (1% v/v) and low (0.01% v/v) odours. The same protocol was followed for blocks where the interleaved lower concentrations were 0.1 and 0.25% v/v (for example, Fig. 4c ). In total, mice were trained on 0.01% v/v odours for 30 blocks, 0.1% v/v odours for 20 blocks and 0.01% for 20 blocks, and 0.25% v/v odours for 7 blocks. Mice were trained to discriminate an odour pair (for example, pair A) until they reached criterion and thereafter for a further 40–50 blocks. They were then trained to discriminate a second odour pair (for example, pair B) comprising two novel odours. Once they had reached criterion on odour pair B, they were presented with a recognition test consisting of a further 5 blocks, each comprising 16 pair B odour trials (8 S+ and 8 S−) pseudo-randomly interleaved with four pair A odour trials (that is, recognition test odours; two unrewarded S+ and two S− trials) ( Supplementary Fig. S2c ). The recognition test S+ odour was unrewarded to ensure that mice could not rapidly relearn to discriminate odour pair A. Nasal flush At least 1 day before treatment, mice were given free access to water. Animals were anaesthetized with isoflurane (Abbott Laboratories, UK) and each naris was flushed separately with 3 μl of either NaCl (9%, 263 mOsm, sham) or ZnSO 4 (8.4% ZnSO 4 , 275 mOsm) using a micropipette (Gilson, USA). This was repeated two more times in immediate succession such that mice received a total of three flushes per nares within 5 min. Mice treated with the high-dose ZnSO 4 were subject to a second ZnSO 4 treatment of a further three flushes per nares within 24 h. All mice were allowed at least 24 h to recover after the last nasal flush before returning to water restriction. Data analysis Images were first 2 × 2 binned (WinMix BlockConverter, Optical Imaging Ltd, USA), then those frames recorded during stimulus presentation (frames 35–65) were divided by the average of prestimulus baseline frames 0–25 ( Supplementary Fig. S3c ), providing image stacks that revealed odour-evoked changes in light reflection, that have been shown to correlate with increases in glomerular activity in the olfactory bulb [28] , [41] , [60] . Image stacks from all activity maps were aligned to the first map recorded in session one using software custom written in Matlab (Mathworks, USA) and Labview (NI) ( Supplementary Fig. S4a ). Using ImageJ (NIH, Bethesda), circular ROIs 75 μm in diameter [60] , Supplementary Fig. S4b ) were positioned over areas with odour-evoked signal in the first activity map recorded in session one during presentation of 1% v/v odours. The same set of ROIs was imposed upon aligned images from all activity maps of all sessions and concentrations for a particular odour and for a particular olfactory bulb. For each image frame, all pixel intensity values were normalized by dividing by the average pixel intensity of the whole image. The mean normalized pixel value of each ROI was then determined and averaged over 40 stimulus frames (frames 10–50 after odour onset) and subtracted from 1. Pixel intensity values for each ROI were correlated with the concomitant ROI recorded in other activity maps recorded in the same bulb for the same odour. All ROI correlations for a given activity map were then averaged, yielding an r -value for each activity map comparison ( Supplementary Fig. S4c ). Across-session correlations were subtracted from within-session correlations, yielding a dissimilarity score whereby high scores indicate large differences between session one and session two odour-evoked activity maps. For determining relative ROI intensities, activity maps that had within-session correlation coefficient r -values lower than 0.5 and ROIs whose normalized average pixel intensity did not on average drop below 0.9990 during odour presentation in both sessions one and two, were removed to ensure that only those ROIs that contained signal in both session were included in analyses. The number of ROIs removed from activity maps of sham and low-dose-ZnSO 4 -treated mice following thresholding was not significantly different (median of ratio of number of ROIs before filtering to after filtering, sham, 1.83±1.5, n =15 activity maps, low-dose-ZnSO 4 -treated, 2.71±1.3, n =9 activity maps, P >0.1). For activity maps recorded at different concentrations, the mean ratio of number of ROIs obtained from activity maps evoked by lower concentrations in session two were not significantly different from the ratio obtained from 1% v/v presented in both sessions (1% v/v session one versus 1% v/v session two, median ratio, 1±0.278, n =7; session two, 0.1% v/v, median ratio, 1.65±1.27, n =5, P >0.1; session two, 0.05% v/v, median ratio 1.19±0.67, n =7, P >0.1; session two, 0.01% v/v, median ratio, 1.57±0.89, n =7, P >0.1). After thresholding, intensity values of each ROI were averaged across blocks and then ranked. Session two ROIs were ordered according to their rank in session one. ROI intensity values for session one and two were then normalized to 1 and session two values were subtracted from session one values to determine the extent of change in relative ROI intensity across sessions for the whole activity map. Subtraction values for all ROIs were then compiled and the population statistics determined. A higher variance of subtraction values indicated a higher change in relative intensity. ROI intensity subtraction values were compared using Ansari Bradley tests after subtracting medians. Dissimilarity scores were compared using Mann–Whitney’s U -tests. How to cite this article: Bracey, E. F. et al . Perceptual judgements and chronic imaging of odour maps indicate comprehensive stimulus template matching in olfaction. Nat. Commun. 4:2100 doi: 10.1038/ncomms3100 (2013).